Fucose-specific DC-SIGN signalling directs T helper cell type-2 responses via IKKε- and CYLD-dependent Bcl3 activation Carbohydrate-specific signalling through DC-SIGN provides dendritic cells with plasticity to tailor immunity to the nature of invading microbes. Here we demonstrate that recognition of fucose-expressing extracellular pathogens like Schistosoma mansoni and Helicobacter pylori by DC-SIGN favors T helper cell type-2 (T H 2) responses via activation of atypical NF-κB family member Bcl3. Crosstalk between TLR and DC-SIGN signalling results in TLR-induced MK2-mediated phosphorylation of LSP1, associated with DC-SIGN, upon fucose binding. Subsequently, IKKε and CYLD are recruited to phosphorylated LSP1. IKKε activation is pivotal for suppression of CYLD deubiquitinase activity and subsequent nuclear translocation of ubiquitinated Bcl3. Bcl3 activation represses TLR-induced proinflammatory cytokine expression, while enhancing interleukin-10 (IL-10) and T H 2-attracting chemokine expression, shifting T H differentiation from T H 1 to T H 2 polarization. Thus, DC-SIGN directs adaptive T H 2 immunity to fucose-expressing pathogens via an IKKε-CYLD-dependent signalling pathway leading to Bcl3 activation, which might be targeted in vaccination strategies or to prevent aberrant inflammation and allergy. Dendritic cells (DCs) are not only involved in antigen presentation but are also crucial in initiating specific adaptive immune responses to invading pathogens [1] , [2] . Recognition of pathogens is mediated by pattern recognition receptors (PRRs) that trigger innate signalling to activate DCs. DCs express a plethora of intracellular and extracellular PRRs to deal with the diverse nature of microbes. Fine-tuning of innate signalling by these PRRs is of crucial importance to orchestrate tailor-made responses to distinct pathogens [3] , [4] . T helper (T H ) cell differentiation is driven by cytokine secretion and cell surface expression of co-stimulatory molecules by DCs in response to infectious pathogens; different adaptive responses in the form of T H 1, T helper cell type-2 (T H 2), T H 17, T H 9 and T FH subsets and regulatory T cells support the immune system in appropriately dealing with infectious agents, such as bacteria, viruses, parasites and fungi [5] , [6] . A significant level of plasticity is required from DCs to mount tailor-made responses and different levels of fine-tuning have been described. Foremost, crosstalk between innate signalling pathways induced by PRRs recognizing different pathogen-associated molecular patterns (PAMPs) on microorganisms determines the overall adaptive response [7] , [8] . Innate signalling by Toll-like receptors (TLRs) can be modulated by other PRRs such as C-type lectin receptors (CLRs) and RIG-I-like receptors, dictating the final outcome [4] , [8] , [9] . The CLR DC-SIGN senses the presence of pathogens through recognition of glycans [9] , [10] . We have recently shown that DC-SIGN has the unique ability among PRRs to induce distinct signalling pathways to different pathogens based on the carbohydrates expressed on their PAMPs by switching its ‘signalosome’ [11] . Hence, carbohydrate-specific signalling by DC-SIGN affects the immunological outcome. We have demonstrated that DC-SIGN is constitutively bound by adaptor protein LSP1 in combination with a triad ‘signalosome’ complex consisting of adaptor proteins KSR1 and CNK and kinase Raf-1. Upon recognition of mannose-carrying PAMPs expressed by Mycobacterium tuberculosis and viruses such as HIV-1 by DC-SIGN, this signalosome serves as a docking site for recruited signalling proteins that activate Raf-1 (ref. 11 ). Raf-1-dependent signalling modulates TLR-induced NF-κB activation via phosphorylation and acetylation of NF-κB subunit p65, which enhances proinflammatory cytokine expression, thus fine-tuning the instigated immune response [11] , [12] . In contrast, upon recognition of fucose-carrying pathogens such as the human gastric bacteria Helicobacter pylori by DC-SIGN, the KSR1-CNK-Raf-1 signalosome is displaced from the cytoplasmic tail of DC-SIGN, while LSP1 remains attached. Fucose-specific DC-SIGN signalling then suppresses proinflammatory responses initiated by TLR4 (ref. 11 ); however, the mechanisms behind these responses remain unknown. A common feature of fucose-expressing pathogens such as H. pylori and also helminth parasites such as Schistosoma mansoni is their ability to inhibit T H 1 responses [13] or even drive T H differentiation towards T H 2 responses [14] , [15] . Several studies suggest that recognition of fucose PAMPs on these pathogens by DC-SIGN is involved in adaptive immune responses [11] , [13] , [15] ; however, it remains elusive whether these pathogens use similar routes to induce T H 2 responses or whether other routes exist and/or contribute. Here we have identified the innate signalling pathways triggered by recognition of fucose ligands by DC-SIGN that lead to the suppression of proinflammatory cytokines and induction of T H 2 polarization. We show that DC-SIGN binding to fucose-expressing PAMPs from S. mansoni and H. pylori induces signalling that intersects with TLR signalling leading to phosphorylation of LSP1, subsequently allowing recruitment of IKKε and CYLD to LSP1. CYLD activity constitutively keeps the atypical NF-κB family member Bcl3 in the cytoplasm, but IKKε-dependent deactivation of CYLD by fucose-specific triggering of DC-SIGN results in nuclear accumulation of Bcl3. Nuclear Bcl3 subsequently forms complexes with p50 homodimers, interfering with p65–p50 binding and modulating TLR-induced cytokine expression; Bcl3–p50 complexes upregulate IL-10 and the T H 2-attracting chemokines CCL17 and CCL22, while downregulating IL-12, and shifting T H differentiation from a T H 1 towards a T H 2 response. Thus, crosstalk between TLRs and DC-SIGN drives T H 2 immunity to fucose-carrying pathogens through IKKε-dependent Bcl3 activation. Fucose-DC-SIGN modulates cytokine responses via Bcl3 Fucose-containing DC-SIGN ligand Lewis X (LeX) enhanced LPS-induced IL-10 expression in a DC-SIGN- and LSP1-dependent manner ( Fig. 1 ). We have previously shown that LeX binding to DC-SIGN suppresses LPS-induced IL-12p70 and IL-6 expression by DCs [11] ; here we show that IL-23 expression was also decreased by LeX-induced signalling in a DC-SIGN-dependent manner ( Fig. 1a ). Triggering of DC-SIGN alone by LeX did not result in any cytokine production ( Fig. 1a ). IL-12p70 and IL-23 share their IL-12p40 subunit, which dimerizes with IL-12p35 and IL-23p19, respectively [16] . LPS-induced expression of all three subunits was decreased by LeX at the transcriptional level, while blocking DC-SIGN by antibodies or silencing LSP1 by RNA interference ( Supplementary Fig. 1 ) restored expression to levels observed with LPS alone ( Fig. 1b,c ). 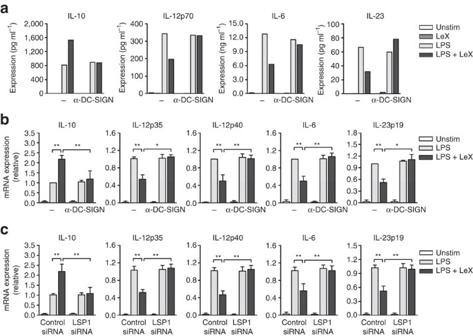Figure 1: Fucose-specific DC-SIGN signalling upregulates IL-10 and downregulates proinflammatory cytokine responses via LSP1. (a) Cytokine secretion in supernatants of DCs 24 h after stimulation with LPS and/or LeX, in the absence or presence of blocking DC-SIGN antibodies, measured by ELISA. (b,c) Cytokine mRNA expression by DCs 6 h after stimulation with LPS and/or LeX, in the absence or presence of blocking DC-SIGN antibodies (b) or after LSP1 silencing (c) by siRNA, measured by real-time PCR, normalized to GAPDH and set at 1 in LPS-stimulated cells. **P<0.01, *P<0.05 (Student’st-test). Data are representative of two (a), at least eight (b) or fifteen (c) independent experiments (mean and s.d. inb,c). Figure 1: Fucose-specific DC-SIGN signalling upregulates IL-10 and downregulates proinflammatory cytokine responses via LSP1. ( a ) Cytokine secretion in supernatants of DCs 24 h after stimulation with LPS and/or LeX, in the absence or presence of blocking DC-SIGN antibodies, measured by ELISA. ( b , c ) Cytokine mRNA expression by DCs 6 h after stimulation with LPS and/or LeX, in the absence or presence of blocking DC-SIGN antibodies ( b ) or after LSP1 silencing ( c ) by siRNA, measured by real-time PCR, normalized to GAPDH and set at 1 in LPS-stimulated cells. ** P <0.01, * P <0.05 (Student’s t -test). Data are representative of two ( a ), at least eight ( b ) or fifteen ( c ) independent experiments (mean and s.d. in b , c ). Full size image Transcriptional regulation of cytokine gene expression is largely regulated through family members of transcription factor NF-κB [17] , [18] . We found that LeX triggering did not affect activation and nuclear translocation of NF-κB subunit p65 by LPS ( Fig. 2a ). We therefore performed chromatin immunoprecipitation (ChIP) assays to directly investigate the binding of p50–p65 dimers to the transcription regulatory regions of IL-10 , IL-12A , IL-12B , IL-23A and IL-6 . p50 homodimers were bound to all genes in unstimulated DCs ( Fig. 2b ), keeping transcription of these genes silent in immature DCs, due to their lack of a transactivation domain [18] , [19] . We observed that both p50 and p65 were bound to NF-κB binding sites of cytokine genes in LPS-stimulated DCs ( Fig. 2b ). Notably, p65 was almost completely absent after LPS/LeX costimulation, whereas p50 was still present ( Fig. 2b ). These data indicate that formation of p50-p65 dimers or their binding to transcription regulatory regions within the nucleus is disturbed due to DC-SIGN signalling via LeX. We hypothesized that another factor interferes with p50–p65 binding, allowing p50–p50 binding and conferring either transactivating or inhibitory properties to the p50 homodimer in a context-specific manner. An atypical member of the NF-κB family is Bcl3, which can associate with p50 homodimers to form Bcl3–p50–p50 complexes [18] . Bcl3 has been reported to be involved in restricting inflammation by both suppressing IL-23 and inducing IL-10 (refs 17 , 20 , 21 ). To establish whether Bcl3 plays a role in fucose-specific DC-SIGN signalling, we performed re-ChIP experiments in which we did a second immunoprecipitation (IP) with Bcl3, p65 or p50 antibodies on DNA-p50 or DNA-p65 complexes. The IL 10 , IL 12A , IL 12B , IL 23A and IL 6 genes were occupied by p50-p65 dimers after LPS stimulation ( Fig. 2c ). Remarkably, after LPS/LeX costimulation, the NF-κB sites were primarily bound by p50 associated with Bcl3 ( Fig. 2c ). These results strongly suggest that Bcl3 plays a primary role in the fucose-specific modulation of TLR-induced cytokine response by DC-SIGN. 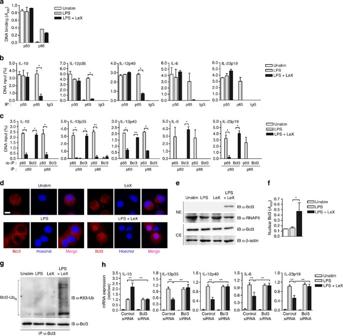Figure 2: Fucose-specific DC-SIGN signalling modulates cytokine responses via Bcl3. (a) NF-κB subunit activation in nuclear extracts of DCs 2 h after stimulation with LPS and/or LeX, measured by DNA binding ELISA. (b,c) p65 and p50 recruitment to NF-κB binding motifs of cytokine gene regulatory regions in DCs 2 h after stimulation with LPS and/or LeX, determined by ChIP assay. IgG indicates a negative control. (c) re-ChIP analysis of the samples shown inbto establish p65–p50, p50-Bcl3 or p65-Bcl3 complex recruitment. Data are expressed as % input DNA. **P<0.01, *P<0.05 (Student’st-test). (d–f) Nuclear translocation of Bcl3 in DCs 2 h after stimulation with LPS and/or LeX, determined by immunofluorescence microscopy (d; Bcl3, red; Hoechst staining, blue; merge, pink; scale bar, 10 μm), IB (e; nuclear, NE; cytoplasmic, CE extracts) or ELISA (f). Ine, RNAPII and β-actin served as loading controls for NE and CE, respectively. *P<0.05 (Student’st-test). See alsoSupplementary Fig. 5. (g) K63-linked polyubiquitination (K63-Ub) of Bcl3 in whole-cell lysates of DCs 2 h after stimulation with LPS and/or LeX, determined by IB after Bcl3 IP. See alsoSupplementary Fig. 5. (h) Cytokine mRNA expression by DCs 6 h after stimulation with LPS and/or LeX, after Bcl3 silencing, measured by real-time PCR, normalized to GAPDH and set at 1 in LPS-stimulated cells. **P<0.01 (Student’st-test). Data are representative of two (a–d,g), five (e), four (f) or at least six (h) independent experiments (mean and s.d. ina–c,f,h). Figure 2: Fucose-specific DC-SIGN signalling modulates cytokine responses via Bcl3. ( a ) NF-κB subunit activation in nuclear extracts of DCs 2 h after stimulation with LPS and/or LeX, measured by DNA binding ELISA. ( b , c ) p65 and p50 recruitment to NF-κB binding motifs of cytokine gene regulatory regions in DCs 2 h after stimulation with LPS and/or LeX, determined by ChIP assay. IgG indicates a negative control. ( c ) re-ChIP analysis of the samples shown in b to establish p65–p50, p50-Bcl3 or p65-Bcl3 complex recruitment. Data are expressed as % input DNA. ** P <0.01, * P <0.05 (Student’s t -test). ( d – f ) Nuclear translocation of Bcl3 in DCs 2 h after stimulation with LPS and/or LeX, determined by immunofluorescence microscopy ( d ; Bcl3, red; Hoechst staining, blue; merge, pink; scale bar, 10 μm), IB ( e ; nuclear, NE; cytoplasmic, CE extracts) or ELISA ( f ). In e , RNAPII and β-actin served as loading controls for NE and CE, respectively. * P <0.05 (Student’s t -test). See also Supplementary Fig. 5 . ( g ) K63-linked polyubiquitination (K63-Ub) of Bcl3 in whole-cell lysates of DCs 2 h after stimulation with LPS and/or LeX, determined by IB after Bcl3 IP. See also Supplementary Fig. 5 . ( h ) Cytokine mRNA expression by DCs 6 h after stimulation with LPS and/or LeX, after Bcl3 silencing, measured by real-time PCR, normalized to GAPDH and set at 1 in LPS-stimulated cells. ** P <0.01 (Student’s t -test). Data are representative of two ( a – d , g ), five ( e ), four ( f ) or at least six ( h ) independent experiments (mean and s.d. in a – c , f , h ). Full size image Bcl3 resides primarily in the cytoplasm in resting DCs, while K63-linked Bcl3 polyubiquitination appears to induce its translocation from the cytoplasm to the nucleus, where it associates with p50-p50 or p52-p52 (refs 18 , 22 ). We next investigated whether DC-SIGN triggering by LeX alone or in combination with LPS induces Bcl3 nuclear translocation. Notably, nuclear translocation of Bcl3 was only observed with simultaneous LPS/LeX stimulation, while neither TLR4 nor DC-SIGN triggering alone activated Bcl3 ( Fig. 2d–f ). Furthermore, LPS/LeX costimulation enhanced K63-linked polyubiquitination of Bcl3, compared with either LPS or LeX stimulation alone ( Fig. 2g ). Moreover, Bcl3 silencing ( Supplementary Fig. 1 ) completely abrogated LeX-mediated modulation of LPS-induced cytokine responses, without affecting TLR4 signalling ( Fig. 2h ). These data show that fucose-specific signalling by DC-SIGN results in activation and nuclear localization of Bcl3, where it cooperates with p50 and interferes with p65–p50 binding to modulate cytokine gene expression. Furthermore, unlike Raf-1 kinase activation by mannose-specific DC-SIGN ligands [11] , [12] , fucose-mediated Bcl3 activation requires crosstalk between TLR4 and DC-SIGN signalling. Bcl3 is activated via IKKε activation and CYLD inactivation Nuclear translocation of Bcl3 is prevented by the continuous removal of its K63-linked polyubiquitin chains by deubiquitinase (DUB) CYLD [22] . CYLD DUB activity is decreased by phosphorylation of CYLD at Ser418, a process mediated by noncanonical IKK kinase family member IKKε [23] . We investigated whether CYLD phosphorylation and activity were affected by DC-SIGN signalling. We observed that CYLD was phosphorylated at Ser418 in DCs stimulated with LPS/LeX in contrast to LeX or LPS alone ( Fig. 3a,b ). Although CYLD was constitutively active in unstimulated DCs and LPS treatment did not affect its DUB activity, LPS/LeX stimulation significantly reduced its DUB activity, but did not completely abrogate its activity ( Fig. 3c ). Furthermore, blocking DC-SIGN signalling by silencing of LSP1 abrogated CYLD Ser418 phosphorylation and restored its impaired DUB activity ( Fig. 3b,c ). Notably, IKKε silencing ( Supplementary Fig. 1 ) also prevented CYLD phosphorylation at Ser418 and subsequent decrease in its DUB activity after LPS/LeX costimulation ( Fig. 3b,c ), indicating that IKKε plays a role in fucose-dependent DC-SIGN signalling. Silencing of CYLD expression ( Supplementary Fig. 1 ) resulted in nuclear accumulation of Bcl3 in unstimulated DCs ( Supplementary Fig. 2 ), consistent with its role in controlling Bcl3 activation. However, cytokine expression was significantly enhanced in LPS-stimulated CYLD-silenced DCs ( Supplementary Fig. 2 ), despite this nuclear Bcl3 accumulation, while costimulation with LeX had no further effects ( Supplementary Fig. 2 ). CYLD has an important role in restricting immune responses from turning into excessive inflammation by negatively regulating NF-κB activation via TAK1 deubiquitination [24] , [25] . Our data suggest that complete CYLD inhibition via CYLD silencing in DCs leads to p65 hyperactivation, which predominates over nuclear Bcl3 effects, hence leading to activation of cytokine responses, in contrast to the restricted CYLD inactivation induced via DC-SIGN that leads to Bcl3-mediated suppression of cytokine transcription ( Fig. 1 ), without inducing p65 hyperactivation ( Fig. 2a ). 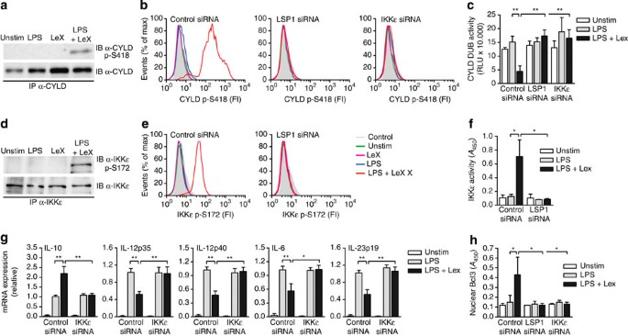Figure 3: DC-SIGN-mediated Bcl3 activation requires IKKε activation and CYLD deactivation. (a,b,d,e) CYLD phosphorylation at Ser418 (a,b) or IKKε phosphorylation at Ser172 (d,e) in DCs left unstimulated (green) or 30 min after stimulation with LeX (pink), LPS (blue) or LPS/LeX (red), after LSP1 or IKKε silencing, determined by IB (a,d; IP) or flow cytometry (b,e; FI, fluorescence intensity). See alsoSupplementary Fig. 6. (c,f) CYLD DUB or IKKε kinase activity in whole-cell lysates of DCs 30 min after stimulation with LPS and/or LeX, after LSP1 or IKKε silencing. **P<0.01, *P<0.05 (Student’st-test). (g) Cytokine mRNA expression by DCs 6 h after stimulation with LPS and/or LeX, after IKKε silencing, measured by real-time PCR, normalized to GAPDH and set at 1 in LPS-stimulated cells. **P<0.01 (Student’st-test). (h) Bcl3 expression in nuclear extracts of DCs 2 h after stimulation with LPS and/or LeX, after LSP1 or IKKε silencing, measured by ELISA. *P<0.05 (Student’st-test). Data are representative of two (a,b,d,e), four (c), three (f,h) or at least five (g) independent experiments (mean and s.d. inc,f,g,h). Figure 3: DC-SIGN-mediated Bcl3 activation requires IKKε activation and CYLD deactivation. ( a , b , d , e ) CYLD phosphorylation at Ser418 ( a , b ) or IKKε phosphorylation at Ser172 ( d , e ) in DCs left unstimulated (green) or 30 min after stimulation with LeX (pink), LPS (blue) or LPS/LeX (red), after LSP1 or IKKε silencing, determined by IB ( a , d ; IP) or flow cytometry ( b , e ; FI, fluorescence intensity). See also Supplementary Fig. 6 . ( c , f ) CYLD DUB or IKKε kinase activity in whole-cell lysates of DCs 30 min after stimulation with LPS and/or LeX, after LSP1 or IKKε silencing. ** P <0.01, * P <0.05 (Student’s t -test). ( g ) Cytokine mRNA expression by DCs 6 h after stimulation with LPS and/or LeX, after IKKε silencing, measured by real-time PCR, normalized to GAPDH and set at 1 in LPS-stimulated cells. ** P <0.01 (Student’s t -test). ( h ) Bcl3 expression in nuclear extracts of DCs 2 h after stimulation with LPS and/or LeX, after LSP1 or IKKε silencing, measured by ELISA. * P <0.05 (Student’s t -test). Data are representative of two ( a , b , d , e ), four ( c ), three ( f , h ) or at least five ( g ) independent experiments (mean and s.d. in c , f , g , h ). Full size image The mechanisms leading to IKKε activation are poorly defined; however, activation of its kinase activity requires phosphorylation at Ser172 within the activation loop [26] , [27] . We found that IKKε became phosphorylated at Ser172 after combined LPS/LeX stimulation, but not LPS or LeX stimulation alone ( Fig. 3d,e ), consistent with the requirement for both signalling pathways in IKKε-mediated CYLD phosphorylation ( Fig. 3a,b ). Furthermore, IKKε phosphorylation after LPS/LeX treatment resulted in activation of its kinase activity, in a LSP1-dependent, but CYLD-independent manner ( Fig. 3e,f and Supplementary Fig. 2 ). IKKε activation was crucial in fucose-dependent cytokine responses as IKKε silencing prevented LeX-mediated modulation of LPS-induced cytokine responses ( Fig. 3g ). These results strongly suggest that crosstalk between TLR4 and fucose-induced DC-SIGN signalling leads to IKKε activation and subsequent deactivation of CYLD, thereby resulting in modulation of LPS-induced cytokine responses via Bcl3. Indeed, silencing of either LSP1 or IKKε abrogated the nuclear accumulation of Bcl3 observed in DCs stimulated with LPS/LeX ( Fig. 3h ). IKKε-CYLD associate with DC-SIGN after LSP1 phosphorylation We next investigated whether LeX signalling leads to recruitment of IKKε and CYLD to DC-SIGN. As expected, LSP1 immunoprecipitated together with DC-SIGN from whole-cell extracts of untreated, LPS-, LeX- and LPS/LeX-stimulated DCs ( Fig. 4a ). Notably, both Ser172-phosphorylated IKKε and Ser418-phosphorylated CYLD associated with DC-SIGN only after simultaneous TLR4 and DC-SIGN triggering, but neither after LPS nor LeX stimulation alone ( Fig. 4a ). The association of LSP1 with DC-SIGN is a prerequisite for both IKKε and CYLD recruitment to DC-SIGN as both proteins failed to immunoprecipitate together with DC-SIGN from extracts of LSP1-silenced cells ( Fig. 4b ). These data strongly suggest that DC-SIGN-mediated Bcl3 activation is the result of the recruitment of a ‘fucose signalosome’ consisting of IKKε and CYLD to DC-SIGN via LSP1. 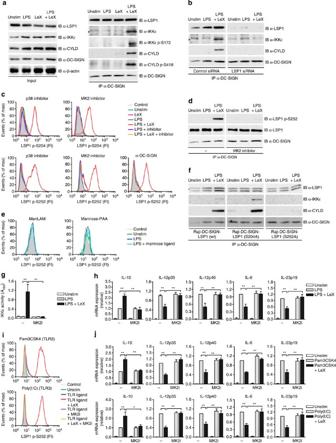Figure 4: IKKε and CYLD recruitment to DC-SIGN requires LSP1 phosphorylation. (a,b,d) LSP1, Ser252-phosphorylated LSP1, IKKε (indicated with >), Ser172-phosphorylated IKKε, CYLD and Ser418-phosphorylated CYLD in whole-cell lysates of DCs 30 min after stimulation with LPS and/or LeX, without (a) or with (b) LSP1 silencing, or in the absence or presence of MK2 inhibitor (d), prior to (input) or after being immunoprecipitated together with DC-SIGN (IP), determined by IB. Ina, β-actin served as loading control. See alsoSupplementary Figs 7–9. (c,e,i) LSP1 phosphorylation at Ser204 (c) and Ser252 (c,e,i) in DCs left unstimulated (green) or 20 min after stimulation with LeX (pink), TLR ligand (blue; LPS, TLR4 ligand; Pam3CSK, TLR2 ligand; poly(I:C), TLR3 ligand), TLR ligand/LeX (red) or TLR ligand plus indicated mannose-based DC-SIGN ligand (cyan), in the absence or presence (TLR ligand, purple; TLR ligand/LeX, orange) of p38 inhibitor (c), MK2 inhibitor (c,i) or blocking DC-SIGN antibodies (c), determined by flow cytometry (FI, fluorescence intensity). (f) LSP1, IKKε and CYLD immunoprecipitated together with DC-SIGN (IP) from whole-cell lysates of Raji-DC-SIGN cells transduced with either GFP-tagged wild-type LSP1 or LSP1 S204A and S252A mutants, 20 min after stimulation with LPS and/or LeX, determined by IB. * indicates GFP-tagged LSP1, while the lower band is endogenous LSP1. See alsoSupplementary Fig. 10. (g) IKKε kinase activity in whole-cell lysates of DCs 30 min after stimulation with LPS and/or LeX, in the absence or presence of MK2 inhibitor. **P<0.01, *P<0.05 (Student’st-test). (h,j) Cytokine mRNA expression by DCs 6 h after stimulation with TLR ligand and/or LeX, in the absence or presence of MK2 inhibitor, measured by real-time PCR, normalized to GAPDH and set at 1 in TLR ligand-stimulated cells. **P<0.01, *P<0.05 (Student’st-test). Data are representative of four (a,b), six (cp-S252), two (cp-S204,d,e,i), one (f), five (g) or at least four (h,j) independent experiments (mean and s.d. ing,h,j). Figure 4: IKKε and CYLD recruitment to DC-SIGN requires LSP1 phosphorylation. ( a , b , d ) LSP1, Ser252-phosphorylated LSP1, IKKε (indicated with >), Ser172-phosphorylated IKKε, CYLD and Ser418-phosphorylated CYLD in whole-cell lysates of DCs 30 min after stimulation with LPS and/or LeX, without ( a ) or with ( b ) LSP1 silencing, or in the absence or presence of MK2 inhibitor ( d ), prior to (input) or after being immunoprecipitated together with DC-SIGN (IP), determined by IB. In a , β-actin served as loading control. See also Supplementary Figs 7–9 . ( c , e , i ) LSP1 phosphorylation at Ser204 ( c ) and Ser252 ( c , e , i ) in DCs left unstimulated (green) or 20 min after stimulation with LeX (pink), TLR ligand (blue; LPS, TLR4 ligand; Pam3CSK, TLR2 ligand; poly(I:C), TLR3 ligand), TLR ligand/LeX ( red ) or TLR ligand plus indicated mannose-based DC-SIGN ligand (cyan), in the absence or presence (TLR ligand, purple; TLR ligand/LeX, orange) of p38 inhibitor ( c ), MK2 inhibitor ( c , i ) or blocking DC-SIGN antibodies ( c ), determined by flow cytometry (FI, fluorescence intensity). ( f ) LSP1, IKKε and CYLD immunoprecipitated together with DC-SIGN (IP) from whole-cell lysates of Raji-DC-SIGN cells transduced with either GFP-tagged wild-type LSP1 or LSP1 S204A and S252A mutants, 20 min after stimulation with LPS and/or LeX, determined by IB. * indicates GFP-tagged LSP1, while the lower band is endogenous LSP1. See also Supplementary Fig. 10 . ( g ) IKKε kinase activity in whole-cell lysates of DCs 30 min after stimulation with LPS and/or LeX, in the absence or presence of MK2 inhibitor. ** P <0.01, * P <0.05 (Student’s t -test). ( h , j ) Cytokine mRNA expression by DCs 6 h after stimulation with TLR ligand and/or LeX, in the absence or presence of MK2 inhibitor, measured by real-time PCR, normalized to GAPDH and set at 1 in TLR ligand-stimulated cells. ** P <0.01, * P <0.05 (Student’s t -test). Data are representative of four ( a , b ), six ( c p-S252), two ( c p-S204, d , e , i ), one ( f ), five ( g ) or at least four ( h , j ) independent experiments (mean and s.d. in g , h , j ). Full size image Although LeX binding to DC-SIGN is sufficient to displace the ‘mannose signalosome’ KSR1-CNK-Raf-1 from LSP1 (ref. 11 ), recruitment of IKKε and CYLD ( Fig. 4a,b ) and subsequent nuclear Bcl3 accumulation ( Fig. 2d ) required crosstalk between TLR4- and fucose-induced DC-SIGN signalling. To address the requirement for this crosstalk, we investigated a possible role for LSP1 modifications in the recruitment of IKKε and CYLD to DC-SIGN. LSP1 is a known target for mitogen-activated protein kinase-activated protein kinase 2 (MK2), a downstream effector of MAP kinase p38 leading to LSP1 phosphorylation at Ser204 and Ser252 in neutrophils, which affects LSP1 interactions with F-actin [28] , [29] . LPS stimulation alone induced phosphorylation and activation of both p38 and MK2 in DCs, which was unaffected by DC-SIGN triggering via LeX ( Supplementary Fig. 3 ). While LPS or LeX stimulation alone was insufficient to induce LSP1 phosphorylation, LPS/LeX stimulation induced LSP1 phosphorylation at both Ser204 and Ser252 in a p38/MK2- as well as DC-SIGN-dependent manner ( Fig. 4c ). LSP1 associated with DC-SIGN within the ‘fucose signalosome’ was phosphorylated in a MK2-dependent manner ( Fig. 4d ), whereas DC-SIGN triggering with different mannose-based ligands did not induce LSP1 phosphorylation ( Fig. 4e ). These data suggest that prior displacement of the ‘mannose signalosome’ is a prerequisite for LSP1 phosphorylation via the LPS-activated p38/MK2 pathway. To establish whether LSP1 phosphorylation affects recruitment of the IKKε-CYLD ‘fucose signalosome’ to DC-SIGN, we generated Raji cell lines stably expressing DC-SIGN in combination with wild-type LSP1 or LSP1 mutants where either Ser204 or Ser252 had been substituted by alanine residues to block phosphorylation. We observed IP of LSP1, IKKε and CYLD together with DC-SIGN in LPS/LeX-treated Raji-DC-SIGN cells expressing either wild-type LSP1 or LSP1-S204A mutant ( Fig. 4f ). Remarkably, IKKε and CYLD did not associate with DC-SIGN after LPS/LeX stimulation in Raji-DC-SIGN cells expressing the LSP1-S252A mutant ( Fig. 4f ), neither LSP1 mutation interfered with its association with DC-SIGN ( Fig. 4f ). Furthermore, FACS analyses confirmed that Raji-DC-SIGN cells expressing the LSP1-S252A mutant were deficient in Ser252 phosphorylation after LPS/LeX stimulation, while the wild-type LSP1 and LSP1-S204A-mutant cell lines showed normal LSP1 Ser252 phosphorylation in response to TLR4-DC-SIGN triggering ( Supplementary Fig. 3 ). These results show that recruitment of IKKε and CYLD to DC-SIGN depends on LPS-mediated LSP1 phosphorylation at Ser252 via p38/MK2 as well as fucose-specific DC-SIGN triggering. Moreover, MK2 inhibition completely abrogated IKKε kinase activation after LPS/LeX stimulation ( Fig. 4g ) as well as LeX-mediated modulation of LPS-induced cytokine expression ( Fig. 4h ). We next investigated whether triggering of other TLRs also leads to crosstalk with DC-SIGN-fucose signalling. While TLR4 induces signals via both MyD88 and TRIF adaptor proteins, TLR2 signalling depends on MyD88, while TLR3 signalling requires TRIF [8] . We observed that either TLR2 or TLR3 ligation, with Pam3CSK4 and poly(I:C) respectively, induced MK2 activation ( Supplementary Fig. 3 ), which led to MK2-dependent LSP1 Ser252 phosphorylation after either Pam3CSK4/LeX or poly(I:C)/LeX costimulation ( Fig. 4i ). Furthermore, DC-SIGN triggering by LeX-modulated TLR2- and TLR3-induced cytokine responses similar to TLR4-induced cytokine expression, in an MK2-dependent manner ( Fig. 4j ). Thus, crosstalk between MK2-activating PRRs and DC-SIGN signalling results in recruitment of a ‘fucose-specific’ signalosome consisting of IKKε and CYLD to DC-SIGN via Ser252-phosphorylated LSP1, which is essential for the modulation of TLR-induced cytokine responses. Bcl3 mediates expression of T H 2-attracting chemokines Besides low IL-12 expression, other factors are also involved in favoring T H differentiation towards a T H 2 response [5] . The related chemokines CCL17 and CCL22 function as T H 2-attracting molecules [30] . We observed a significant increase in both CCL17 and CCL22 expression by DCs after LPS/LeX costimulation, compared with LPS-induced expression, which was dependent on DC-SIGN triggering ( Fig. 5a ). Remarkably, fucose-induced Bcl3–p50 complexes functioned as positive regulators of CCL17 and CCL22 transcription ( Fig. 5b,c ). Re-ChIP experiments showed that NF-κB sites within the CCL17 and CCL22 promoters were primarily bound by p50-Bcl3 after LPS/LeX stimulation, while only small amounts of p65-50 dimers were detectable on the CCL17 but not the CCL22 promoter, after LPS stimulation alone ( Fig. 5b ). Furthermore, not only Bcl3 silencing, but also LSP1 and IKKε silencing attenuated LPS/LeX-induced CCL17 and CCL22 messenger RNA (mRNA) expression ( Fig. 5c ), indicating that fucose-specific DC-SIGN-mediated activation of Bcl3 via IKKε affects both cytokine and chemokine expression associated with T H 2 differentiation. 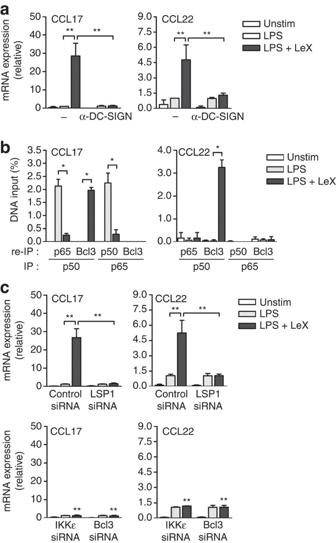Figure 5: IKKε-dependent Bcl3 activation via DC-SIGN induces CCL17 and CCL22 expression. (a,c) Chemokine mRNA expression by DCs 6 h after stimulation with LPS and/or LeX, in the absence or presence of blocking DC-SIGN antibodies (a) or after LSP1, IKKε or Bcl3 silencing (c), measured by real-time PCR, normalized to GAPDH and set at 1 in LPS-stimulated cells. **P<0.01 (Student’st-test). (b) p65–p50, p50-Bcl3 or p65-Bcl3 recruitment to NF-κB binding motifs ofCCL17andCCL22in DCs 2 h after stimulation with LPS and/or LeX, determined by re-ChIP assay. IgG indicates a negative control. Data are expressed as % input DNA. *P<0.05 (Student’st-test). Data are representative of at least four (a), two (b) or three (c) independent experiments (mean and s.d. ina–c). Figure 5: IKKε-dependent Bcl3 activation via DC-SIGN induces CCL17 and CCL22 expression. ( a , c ) Chemokine mRNA expression by DCs 6 h after stimulation with LPS and/or LeX, in the absence or presence of blocking DC-SIGN antibodies ( a ) or after LSP1, IKKε or Bcl3 silencing ( c ), measured by real-time PCR, normalized to GAPDH and set at 1 in LPS-stimulated cells. ** P <0.01 (Student’s t -test). ( b ) p65–p50, p50-Bcl3 or p65-Bcl3 recruitment to NF-κB binding motifs of CCL17 and CCL22 in DCs 2 h after stimulation with LPS and/or LeX, determined by re-ChIP assay. IgG indicates a negative control. Data are expressed as % input DNA. * P <0.05 (Student’s t -test). Data are representative of at least four ( a ), two ( b ) or three ( c ) independent experiments (mean and s.d. in a – c ). Full size image IKKε-mediated Bcl3 activation directs T H 2 polarization We next investigated whether fucose-expressing PAMPs and pathogens drive T H 2 responses via DC-SIGN through IKKε-CYLD-mediated Bcl3 activation. Soluble egg antigen (SEA) derived from the helminth S. mansoni interacts with DC-SIGN via fucose-containing LeX and LDN-F structures, inducing T H 2 polarization both in vitro and in infected individuals [14] , [15] , [31] . S. mansoni triggers several TLRs such as TLR2, TLR3 and TLR4 (refs 32 , 33 , 34 ), that could provide the required signal for MK2-mediated LSP1 phosphorylation. Here we found that S. mansoni SEA alone did not induce cytokine expression, however modulated LPS-induced cytokine expression in a similar manner as LeX; S. mansoni SEA upregulated LPS-induced IL-10 expression, while IL-12p35, IL-12p40, IL-23p19 and IL-6 levels were reduced ( Fig. 6a and Supplementary Fig. 4 ). The modulation of LPS-induced cytokine expression by S. mansoni SEA was abrogated by blocking DC-SIGN antibodies, as well as LSP1, IKKε and Bcl3 silencing ( Fig. 6a ), providing evidence that S. mansoni SEA treatment of DCs targets DC-SIGN to induce the fucose-specific signalling pathway leading to Bcl3 activation and subsequent modulation of TLR cytokine responses. 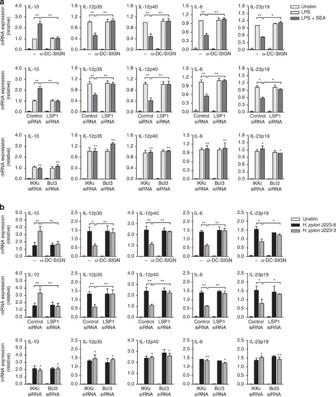Figure 6: Bcl3-mediated modulation of cytokine expression in response to DC-SIGN triggering by fucose PAMPs ofS. mansoniandH. pylori. (a,b) Cytokine mRNA expression by DCs 6 h after stimulation with LPS and/or LeX/LDN-F-positiveS. mansoniSEA (a), LeY-negativeH. pyloriphase-variant J223-8 or LeY-positiveH. pyloriJ223-3 (b), in the absence or presence of blocking DC-SIGN antibodies or after LSP1, IKKε or Bcl3 silencing, measured by real-time PCR, normalized to GAPDH and set at 1 in LPS-stimulated cells. **P<0.01, *P<0.05 (Student’st-test). Data are representative of at least four independent experiments (mean and s.d. ina,b). Figure 6: Bcl3-mediated modulation of cytokine expression in response to DC-SIGN triggering by fucose PAMPs of S. mansoni and H. pylori . ( a , b ) Cytokine mRNA expression by DCs 6 h after stimulation with LPS and/or LeX/LDN-F-positive S. mansoni SEA ( a ), LeY-negative H. pylori phase-variant J223-8 or LeY-positive H. pylori J223-3 ( b ), in the absence or presence of blocking DC-SIGN antibodies or after LSP1, IKKε or Bcl3 silencing, measured by real-time PCR, normalized to GAPDH and set at 1 in LPS-stimulated cells. ** P <0.01, * P <0.05 (Student’s t -test). Data are representative of at least four independent experiments (mean and s.d. in a , b ). Full size image Another known fucose-expressing pathogen for DC-SIGN is H. pylori , which can switch Lewis antigens on LPS on and off through phase-variable expression [13] . H. pylori LPS is recognized by TLR2 (ref. 35 ). While H. pylori strain J223-3 also interacts with DC-SIGN through Lewis Y (LeY), the LeY-negative phase-variant J223-8 does not bind DC-SIGN [13] . We have previously shown that LeY-positive H. pylori J223-3 enhanced IL-10 and decreased IL-12p35, IL-12p40 and IL-6 mRNA expression compared with the LeY-negative strain in a DC-SIGN-dependent manner (ref. 11 and Fig. 6b ). Similarly, we observed lower induction of IL-23p19 mRNA after DC stimulation with LeY-positive H. pylori J223-3 compared with LeY-negative H. pylori J223-8 ( Fig. 6b ). IL-23p19 mRNA expression was restored after H. pylori J223-3 stimulation in the presence of blocking DC-SIGN antibodies ( Fig. 6b ). Furthermore, silencing of LSP1, IKKε and Bcl3 prevented fucose-dependent modulation by LeY-positive H. pylori J223-3 ( Fig. 6b ). Thus, fucose-carrying S. mansoni SEA and phase-variant J223-3 of H. pylori signal via DC-SIGN in a LSP1-IKKε-Bcl3-dependent manner similar to fucose-containing glycoconjugates. We next investigated whether fucose-specific DC-SIGN signalling induces T H 2 immunity to S. mansoni SEA and H. pylori phase variants. We performed T H differentiation assays by coculturing LPS and/or LeX-primed DCs with naive CD4 + T cells and measured intracellular IFNγ and IL-4 expression as markers for T H 1 and T H 2 cells, respectively [36] . Notably, LeX skewed LPS-induced T H differentiation by DCs from a T H 1 response towards a T H 2 response ( Fig. 7a ). Strikingly, inhibition of DC-SIGN signalling by blocking DC-SIGN antibodies as well as by LSP1, IKKε and Bcl3 silencing prevented this T H 2 skewing ( Fig. 7a–c ). Whereas the LeX-expressing PAMP S. mansoni SEA alone did not induce T H proliferation, it skewed LPS-induced T H differentiation towards T H 2 polarization while suppressing T H 1 differentiation, compared with LPS alone, which was dependent on DC-SIGN-LSP1-mediated activation of IKKε and Bcl3 ( Fig. 7a–c ). Priming of DCs with LeY-negative H. pylori phase-variant J223-8 resulted in strong T H 1 polarization, which was unaffected by blocking DC-SIGN antibodies ( Fig. 7d,e ), whereas LeY-positive H. pylori J223-3 induced very strong T H 2 responses ( Fig. 7d ). Inhibition of DC-SIGN signalling by blocking DC-SIGN antibodies or by LSP1, IKKε and Bcl3 silencing completely reversed T H differentiation towards a substantial T H 1 response by H. pylori J223-3-primed DCs ( Fig. 7d–f ). Thus, Bcl3 activation via IKKε-dependent CYLD deactivation is instrumental in the induction of T H 2 polarization and suppression of T H 1 responses after DC-SIGN recognition of fucose structures on extracellular helminthic and bacterial PAMPs. 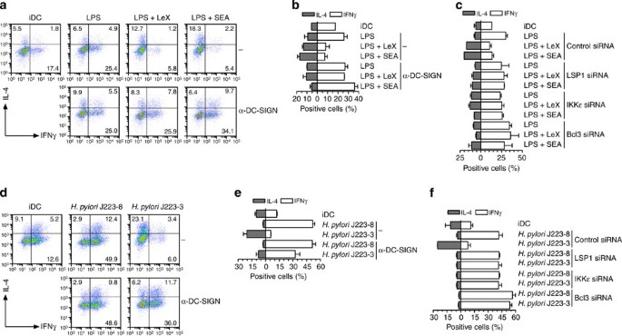Figure 7: DC-SIGN signalling via IKKε and Bcl3 skews T helper cell differentiation towards TH2 polarization in response to fucose-expressing pathogens. (a–f) T helper cell polarization was determined by flow cytometry by staining for intracellular IL-4 (TH2) or IFNγ (TH1) expression after coculture of naive CD4+T cells with DCs that were left unstimulated (iDC) or primed for 48 h with LPS and LeX orS. mansoniSEA (a–c), LeY-negativeH. pyloriphase-variant J223-8 or LeY-positiveH. pyloriJ223-3 (d–f), in the absence or presence of blocking DC-SIGN antibodies (a,b,d,e) or after LSP1, IKKε or Bcl3 silencing (c,f). In (b) and (e), the % IL-4- and IFNγ-producing T cells are shown, corresponding to the upper left and lower right quadrants of (a) and (d), respectively. Data are representative of at least two (a–fpathogens) or four (a–cLeX) independent experiments (mean and s.d. of duplicates inb,c,e,f). Figure 7: DC-SIGN signalling via IKKε and Bcl3 skews T helper cell differentiation towards T H 2 polarization in response to fucose-expressing pathogens. ( a – f ) T helper cell polarization was determined by flow cytometry by staining for intracellular IL-4 (T H 2) or IFNγ (T H 1) expression after coculture of naive CD4 + T cells with DCs that were left unstimulated (iDC) or primed for 48 h with LPS and LeX or S. mansoni SEA ( a – c ), LeY-negative H. pylori phase-variant J223-8 or LeY-positive H. pylori J223-3 ( d – f ), in the absence or presence of blocking DC-SIGN antibodies ( a , b , d , e ) or after LSP1, IKKε or Bcl3 silencing ( c , f ). In ( b ) and ( e ), the % IL-4- and IFNγ-producing T cells are shown, corresponding to the upper left and lower right quadrants of ( a ) and ( d ), respectively. Data are representative of at least two ( a – f pathogens) or four ( a – c LeX) independent experiments (mean and s.d. of duplicates in b , c , e , f ). Full size image Adaptive immune responses that deal adequately and appropriately with invading pathogens depend on strict instructions from DCs and are determined by crosstalk between innate signalling induced via different PRRs upon sensing distinct microbial PAMPs [4] , [7] . Here we identified the molecular mechanism induced via fucose-specific PAMP recognition by DC-SIGN that modulates TLR signalling and instructed T H 2 immunity to extracellular pathogens ( Fig. 8 ). Fucose recognition by DC-SIGN-induced phosphorylation of LSP1 by the TLR-activated p38/MK2 pathway. While the constitutively bound KSR1-CNK-Raf-1 signalosome, required for mannose-specific DC-SIGN signalling, was dissociated from LSP1, phosphorylation of LSP1 allowed recruitment of kinase IKKε and DUB CYLD. IKKε suppressed CYLD activity, which resulted in nuclear accumulation of transcription factor Bcl3. Formation of a Bcl3–p50 complex enhanced the transcriptional activity of IL 10 and chemokines CCL17 and CCL22 , whereas, in contrast, IL-12, IL-23 and IL-6 expression was strongly downregulated, resulting in T H 2 immune responses. The carbohydrate-specific signalling pathways induced via DC-SIGN provide the innate immune system with the molecular means to instruct T cells and induce humoral immunity to fucose-expressing pathogens like S. mansoni and H. pylori . 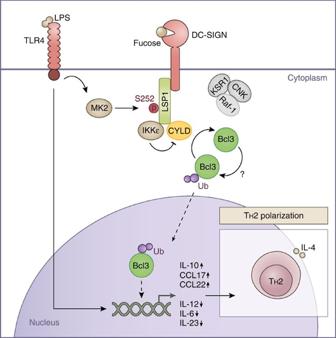Figure 8: Fucose-specific DC-SIGN signalling leads to Bcl3-dependent TH2 differentiation. Binding of fucose ligands to DC-SIGN results in the displacement of the triad signalosome complex KSR1-CNK-Raf-1 from the constitutive DC-SIGN-LSP1 complex. Simultaneous TLR4 triggering by LPS results in the activation of kinase MK2, which leads to the phosphorylation of DC-SIGN-associated LSP1 at Ser252. This crosstalk between TLR-induced MK2 activation and DC-SIGN signalling allows for the recruitment of kinase IKKε and DUB CYLD to the DC-SIGN-LSP1 complex. Activation of IKKε leads to phosphorylation and thereby deactivation of CYLD. Inhibition of CYLD DUB activity leads to the accumulation of ubiquitinated Bcl3 (Bcl3-Ub), which translocates into the nucleus, where it binds to NF-κB subunit p50 present on the transcription regulatory regions of distinct cytokine and chemokine promoters. Bcl3 activity upregulates IL-10 cytokine expression as well as TH2-attracting CCL17 and CCL22 chemokines, while suppressing IL-12, IL-6 and IL-23 expression. The combined shift in expression profile of cytokines and chemokines leads to a shift in THdifferentiation towards TH2 polarization. Figure 8: Fucose-specific DC-SIGN signalling leads to Bcl3-dependent T H 2 differentiation. Binding of fucose ligands to DC-SIGN results in the displacement of the triad signalosome complex KSR1-CNK-Raf-1 from the constitutive DC-SIGN-LSP1 complex. Simultaneous TLR4 triggering by LPS results in the activation of kinase MK2, which leads to the phosphorylation of DC-SIGN-associated LSP1 at Ser252. This crosstalk between TLR-induced MK2 activation and DC-SIGN signalling allows for the recruitment of kinase IKKε and DUB CYLD to the DC-SIGN-LSP1 complex. Activation of IKKε leads to phosphorylation and thereby deactivation of CYLD. Inhibition of CYLD DUB activity leads to the accumulation of ubiquitinated Bcl3 (Bcl3-Ub), which translocates into the nucleus, where it binds to NF-κB subunit p50 present on the transcription regulatory regions of distinct cytokine and chemokine promoters. Bcl3 activity upregulates IL-10 cytokine expression as well as T H 2-attracting CCL17 and CCL22 chemokines, while suppressing IL-12, IL-6 and IL-23 expression. The combined shift in expression profile of cytokines and chemokines leads to a shift in T H differentiation towards T H 2 polarization. Full size image Although DC-SIGN is unable to induce immune responses by itself, its carbohydrate-specific signalling pathways communicate at different levels with signalling of other PRRs [11] , [12] , [37] , [38] . While mannose-specific DC-SIGN signalling intersects with TLR signalling at the level of phosphorylation of LPS-induced p65 via DC-SIGN-activated Raf-1 (ref. 12 ), fucose-specific signalling required crosstalk with TLR signalling at a more proximal point. Here we found that TLR-induced activation of the p38/MK2 pathway led to LSP1 phosphorylation at several serine residues, but only after concomitant DC-SIGN binding by a fucose ligand. Specifically, LSP1 phosphorylation at Ser252 was required to subsequently recruit both IKKε and CYLD to LSP1 at the cytoplasmic domain of DC-SIGN. It is unclear whether the phosphorylated residue is the binding site for either IKKε or CYLD, or whether phosphorylation of LSP1 induces conformational changes within LSP1 that modulate its association with other proteins. The sequence of events leading to the recruitment of IKKε and CYLD to phosphorylated LSP1 remains to be resolved. We propose that the most likely mechanism first involves the dissociation of the ‘mannose signalosome’ from DC-SIGN-LSP1 (ref. 11 ) as a result of conformational changes within DC-SIGN after ligand binding [39] . The displacement of the ‘mannose signalosome’ then enables TLR-activated MK2 to target LSP1 for phosphorylation, possibly due to accessibility. This is in line with our observation that TLR signalling alone, despite inducing MK2 activation, does not result in LSP1 phosphorylation. Dissociation of the KSR1–CNK–Raf-1 complex alone, however, is insufficient to induce ‘fucose signalling’, since mannose triggering of DC-SIGN in Raf-1-silenced cells—which show no binding of KSR1-CNK-Raf-1 to LSP1—simply leads to a block in signalling and leaves LPS-induced cytokine expression undisturbed [11] . These studies together seem to suggest that a DC-SIGN-dependent event, possibly conformational changes, is a prerequisite for MK2-mediated LSP1 phosphorylation. The recruitment of IKKε and CYLD to phosphorylated LSP1 is accompanied by activation of IKKε via Ser172 phosphorylation. Either autophosphorylation or trans -phosphorylation of IKKε has been proposed [26] , [40] and it is conceivable that binding of IKKε to LSP1 or bringing several IKKε molecules into close proximity—since DC-SIGN functions as tetramers [39] —is the trigger for Ser172 phosphorylation. Alternatively, another upstream effector of IKKε, which has been proposed to be a member of the MAP3K or MAP4K subfamily [26] , might also be recruited to the ‘fucose signalosome’, whose identity remains to be established. We observed that the resulting IKKε activation in turn led to phosphorylation and deactivation of DUB CYLD. Like IKKε, CYLD is recruited to DC-SIGN-LSP1, most likely to bring it into close proximity of IKKε. The finding that CYLD plays a role in fucose-specific DC-SIGN signalling, thereby actively steering the direction of the immune response is striking, since CYLD has been assigned an important role in restricting immune responses from turning into excessive inflammation by negatively regulating NF-κB responses [24] , [25] . Here we show that CYLD also has a crucial role in directing pathogen-specific adaptive immunity. The intrinsic role of CYLD in switching off NF-κB responses is not compromised by the restricted inactivation of CYLD as a result of DC-SIGN signalling. Once CYLD activity is attenuated, K63-linked polyubiquitinated Bcl3 is transported into the nucleus, where it targets genes whose transcription is under the control of NF-κB. Bcl3 is an atypical member of the NF-κB family as it possesses no DNA binding activity; however, it contains a well-defined transactivation domain. To modulate NF-κB-regulated transcription, it forms trimeric complexes with either p50 or p52 homodimers [17] , [18] . Whether Bcl3 positively or negatively influences transcription of its target genes depends on the context in which Bcl3 binds and how it interacts with or interferes with binding of transcriptional coactivators. Here we demonstrated that fucose-specific DC-SIGN signalling and Bcl3 activity led to the upregulation of TLR-induced anti-inflammatory IL-10 production and T H 2-attracting chemokines, while proinflammatory cytokines IL-12, IL-23 and IL-6 were downregulated, which is consistent with previous reports on the effects of Bcl3 on IL 10 and IL 23A transcription [20] , [21] . Effective immunity to pathogens requires the induction of T helper cell differentiation. Here we demonstrated that crosstalk between different TLRs and fucose-specific DC-SIGN signalling specifically induced T H 2 immunity via Bcl3 activity. Our data show that recognition of extracellular pathogens like S. mansoni and H. pylori by DC-SIGN via fucose-based PAMPs led to downregulation of T H 1-promoting cytokine IL-12 as well as upregulation of T H 2-attracting chemokines CCL17 and CCL22 and as such drove T H differentiation from T H 1 to T H 2 polarization. Helminths and H. pylori trigger diverse TLRs, besides DC-SIGN via fucose-based PAMPs, which supports the relevance of this mechanism for T H 2 induction to different pathogens. Whether the induced Bcl3-dependent T H 2 polarization is beneficial for host or pathogen likely depends on the nature of the invading microbe. The induction of T H 2 immunity seems to facilitate the persistence of H. pylori infections [41] . In contrast, T H 2 differentiation and humoral immunity are essential for the expulsion of intestinal helminths, eosinophil-mediated killing of parasites and limiting tissue damage [42] , [43] . Nonetheless, identification of the molecular mechanisms leading to T H 2 immunity to these pathogens will provide therapeutic targets to combat the infections. Our data show that DC-SIGN triggering plays an important role in T H 2 differentiation in response to S. mansoni infections, but other mechanisms likely support or reinforce the priming of DCs for T H 2 polarization such as SEA component omega-1, which is also involved in T H 2 polarization via degradation of ribosomal and messenger RNA hence impairing protein synthesis [44] . Besides T H 2 polarization via IL-12 downregulation and chemokine induction, we also observed that the DC-SIGN-induced Bcl3-mediated pathway suppressed TLR-induced IL-23 and IL-6 production. Both IL-23 and IL-6 are crucial cytokines for the induction and maintenance of T H 17 cells [45] . The induction of T H 17 responses is associated with severe forms of schistosomiasis with granulomatous inflammation in host tissues, both in mice and humans, although with relatively low incidence in humans [46] , [47] . S. mansoni SEA has been reported to suppress T H 17 differentiation [48] . Our data suggest that fucose-specific cytokine responses via DC-SIGN also function to dampen pathological T H 17 responses during S. mansoni infections, which might underlie the beneficial effects of parasite extracts in treating Crohn’s disease [49] . Thus, here we have identified a crucial role for IKKε- and CYLD-dependent Bcl3 activation by DC-SIGN that drives the induction of T H differentiation towards T H 2 immunity against fucose-carrying pathogens. This fucose-specific signalling route might be targeted for different vaccine strategies to tailor adaptive immunity to T H 2 and humoral responses. Stimulation and RNA interference of DCs Peripheral blood mononuclear cells were isolated from buffy coats of healthy volunteer blood donors (Sanquin) by a Lymphoprep (Axis-Shield) gradient step and monocytes were subsequently isolated by a Percoll (Amersham) gradient step. Monocytes were differentiated into immature DCs in the presence of 500 U ml −1 IL-4 and 800 U ml −1 GM-CSF (both Invitrogen), and used at day 6 or 7. This study was approved by the Medical Ethics Review Committee of the AMC. Cells were stimulated with 10 ng ml −1 Salmonella typhosa LPS (Sigma), 10 μg ml −1 Pam3CSK4, 10 μg ml −1 poly (I:C) (both from Invivogen), 10 μg ml −1 LeX-PAA, 10 μg ml −1 mannose-PAA (both from Lectinity), 10 μg ml −1 ManLAM from M. tuberculosis (provided by J. Belisle, Colorado State University), Helicobacter pylori phase variants J223-3 and J223-8 (MOI 10; provided by B. Appelmelk, VUmc, Amsterdam), 40 μg ml −1 SEA (provided by E.J. Klaver and I. van Die, VUmc, Amsterdam) prepared from S. mansoni eggs (provided by F. Lewis, Biomedical Research Institute, Rockville, MD) [48] . Cells were preincubated with blocking antibodies or inhibitor for 2 h with 20 μg ml −1 anti-DC-SIGN (AZN-D1; generated ‘in-house’ [50] ), 0.5 μM SB203580 (p38 inhibitor [51] ), 2 μM MK2a inhibitor (MAPKAPK2 inhibitor [52] ; both Calbiochem). DCs were transfected with 25 nM small interfering RNA (siRNA) using transfection reagents DF4 (Dharmacon). At 72 h after transfection, cells were used for experiments. SMARTpool siRNAs used were as follows: LSP1 (M-012640-00), CYLD (M-012640-00), IKKε (M-003723-02), Bcl3 (M-003874-02) and non-targeting siRNA (D-001206-13) as a control (Dharmacon). Silencing of expression was verified by real-time PCR and flow cytometry (ref. 11 and Supplementary Fig. 1 ). Raji-DC-SIGN-LSP1 cell lines LSP1 expression plasmid pCMV6-Entry Myc-DDK-tagged ORF LSP1 was obtained from Origene. LSP1 mutants S204A and S252A were generated using QuikChange II XL site-directed mutagenesis kit (Stratagene) and mutations were verified by sequencing. LSP1 coding sequences were subcloned into lentiviral construct pRRL-cPPT-CMV-X2-PRE-SIN-IRES-eGFP [53] . Viruses were produced in 293T cells (ATCC) and used to transduce Raji-DC-SIGN cells [54] . LSP1 mutant expressing cells were sorted based on GFP expression using a BD Influx cell sorter (BD). Cytokine production Cell culture supernatants were harvested after 24 h of stimulation and IL-10, IL-6 (both Invitrogen), IL-12p70 and IL-23 (both eBioscience) were measured by ELISA (enzyme-linked immunosorbent assay) according to the instructions of the manufacturer. Quantitative real-time PCR mRNA was isolated using mRNA capture kit (Roche), cDNA was synthesized using Reverse Transcriptase Kit (Promega) and PCR amplification was performed in the presence of SYBR green (Applied Biosystems) in an ABI 7500 Fast PCR detection system (Applied Biosystems). Specific primers were designed using Primer Express 2.0 (Applied Biosystems; Supplementary Table 1 ). The C t value is defined as the number of PCR cycles where the fluorescence signal exceeds the detection threshold value. For each sample, the normalized amount of target mRNA N t was calculated from the obtained C t values for both target and GAPDH (glyceraldehyde 3-phosphate dehydrogenase) mRNA with N t =2 C t (GAPDH)− C t (target) . The relative mRNA expression was obtained by setting N t in TLR ligand-stimulated samples at 1 within one experiment and for each donor. NF-κB DNA binding and Bcl3 localization Nuclear and cytoplasmic extracts of DCs were prepared after 2 h of stimulation using NucBuster protein extraction kit (Novagen). NF-κB DNA binding was determined using TransAM NF-κB family kit (Active Motif). Bcl3 was detected using Bcl3 ELISA kit (Antibodies-online.com) or by immunoblotting (IB) with anti-Bcl3 (1:200; sc-185; Santa Cruz Biotechnology), followed by incubation with HRP-conjugated secondary antibody (1:2,500; 21230; Pierce) and ECL detection (Pierce). Membranes were also probed with anti-RNAPII (1:1,000; clone CTD4H8; Millipore) or anti-β-actin (1:2,000; sc-81178; Santa Cruz), followed by HRP-conjugated anti-mouse (1:1,000; sc-2314; Santa Cruz) to ensure equal protein loading among cytoplasmic and nuclear extracts, respectively. Bcl3 localization was further determined by immunofluorescense staining: DCs were stimulated, fixed with 4% paraformaldehyde, then permeabilized with 0.2% (vol/vol) Triton X-100 in PBS and stained with anti-Bcl3 (1:50). Incubation of Alexa Fluor 546-conjugated anti-rabbit (1:250; A10040; Invitrogen) was followed by staining of nuclei with Hoechst (Invitrogen). Bcl3 localization was visualized with a Leica DM LB microscope. ChIP assay ChIP and re-ChIP assays were performed using the ChIP-IT Express Enzymatic Shearing and ChIP-IT Express HT kits (both from Active Motif). Briefly, cells were fixed with 1% (vol/vol) paraformaldehyde after 2 h of stimulation, nuclei were isolated and chromatin DNA fragmented by enzymatic shearing (10 min, 37 °C). Protein–DNA complexes were immunoprecipitated using 4 μg anti-p65 (3034; Cell Signaling), anti-p50 (3035; Cell Signaling) or negative control IgG (53010; Active Motif), and protein G-coated magnetic beads. For re-ChIP analyses, protein–DNA complexes were eluted from beads and desalted using the re-ChIP-IT kit (Active Motif). A second round of IP was performed with anti-p65, anti-p50 or anti-Bcl3 (sc-185X; Santa Cruz). DNA was purified after reversal of crosslinks and real-time PCR reactions were then performed with primer sets spanning NF-κB binding sites ( Supplementary Table 1 ). Primers spanning genomic DNA at cytogenetic location 12 p13.3 (Active Motif) were used as a negative control. To normalize for DNA input, a sample for each condition was taken along which had not undergone IP (‘input DNA’); the results are expressed as % input DNA. Detection of DC-SIGN-fucose signalosome by IB DCs or Raji-DC-SIGN-LSP1 cell lines were stimulated for 30 min and whole-cell extracts were prepared using RIPA Buffer (Cell Signaling). Detection of DC-SIGN-associated proteins was performed by immunoprecipitating DC-SIGN from 40 μg of extract with 4 μg anti-DC-SIGN (AZN-D1) coated on protein A/G-PLUS agarose beads (Santa Cruz). Either 20 μg of extract or immunoprecipitates were resolved by SDS–PAGE, and detected by IB with anti-DC-SIGN (1:500; sc-20081; Santa Cruz), anti-LSP1 (1:2,000; 3812; Cell Signaling), anti-LSP1 p-S252 (1:1,000; ab21636; Abcam), anti-IKKε (1:500; 2905; Cell Signaling), anti-IKKε p-S172 (1:500; 06-1340; Millipore), anti-CYLD (1:500; sc-25779; Santa Cruz) or anti-CYLD p-S418 (1:500; 4500; Cell Signaling), followed by incubation with HRP-conjugated secondary antibody and ECL detection. To ensure equal protein content prior to IP, membranes were also incubated with anti-β-actin, followed by HRP-conjugated anti-mouse. Detection of protein ubiquitination and phosphorylation DCs were stimulated for 30 min (IKKε, CYLD) or 2 h (Bcl3) and whole-cell extracts were prepared as described above. Detection of K63-linked polyubiquitination of Bcl3 was performed by immunoprecipitating Bcl3 from 40 μg of extract with anti-Bcl3 (10 μl; H00000602-PW2; Abnova) coated on protein A/G-PLUS agarose beads (Santa Cruz). Immunoprecipitates were resolved by SDS–PAGE, and detected by IB with anti-Bcl3 (sc-185) or anti-K63-Ub (1:250; 14-6077; Affymetrix), followed by incubation with HRP-conjugated secondary antibody and ECL detection. Phosphorylation of IKKε and CYLD was also detected as described above, after immunoprecitation with 4 μg anti-IKKε or anti-CYLD and IB with anti-IKKε, anti-IKKε p-S172, anti-CYLD and anti-CYLD p-S418. Phosphorylation of IKKε and CYLD (after 30 min stimulation), LSP1, p38 and MK2 (20 min) was further detected by flow cytometry and analysed on a FACS Calibur (BD). Cells were first fixed in 3% paraformaldehyde for 10 min and permeabilized in 90% methanol at 4 °C for 30 min. Primary antibody incubation with anti-LSP1 p-S252 (1:50), anti-LSP1 p-S204 (1:50; MAB0008; Abnova), anti-IKKε p-S172 (1:50), anti-CYLD p-S418 (1:50) and anti-p38 p-T180-Y182 (1:50; 9211; Cell Signaling) was followed by incubation with PE-conjugated anti-rabbit (1:200; 711-116-152; Jackson Immunoresearch). Phosphorylated MK2 was detected with Alexa Fluor 647-conjugated anti-MK2 p-T334 (1:10; 4320; Cell Signaling). IKK ε and CYLD activity assays DCs were stimulated for 30 min and whole-cell extracts were prepared using kinase lysis buffer (50 mM Tris–HCl (pH 7.5), 150 mM NaCl, 1 mM EDTA, 1 mM EGTA, 1 mM DTT, 2 mM Na 3 VO 4 , 1 mM NaF, 50 mM β-glycerophosphate, 1% Triton X-100, 10 μg ml −1 leupeptin, 10 μg ml −1 pepstatin A, 0.4 mM PMSF). Detection of IKKε activity was performed by immunoprecipitating IKKε with 10 μg anti-IKKε (sc-10760; Santa Cruz)-coated protein A/G-PLUS agarose beads from 250 μg of extract. The immunocomplexes were incubated with 1.5 μM biotinylated Pak1(Ser144)/Pak2(Ser141) substrate peptide in kinase buffer with 200 μM ATP (from HTScan IKKε kinase assay kit; Cell Signaling) for 30 min at 30 °C. Biotin-peptide was captured in streptavidin-coated plates (Sigma), and phosphorylation of the peptide was detected using anti-phospho-(Ser/Thr) Phe (9631; Cell Signaling), followed by incubation with HRP-conjugated anti-mouse IgG and assayed using TMB substrate (all from HTScan IKKε kinase assay kit). After termination of the colouring reaction, the absorbance was measured at 450 nm. The level of phosphorylation is a measure for IKKε kinase activity. CYLD activity was measured using DUB-Glo protease assay (Promega) after capturing CYLD in anti-CYLD (sc-25779; Santa Cruz)-coated white-walled high-binding 96-wells plates from 20 μg of extract. The detected relative light units are a measure for CYLD DUB activity. T cell differentiation assay Naive CD4 + T cells were isolated using CD4 + T cell isolation kit II (Miltenyi), combined with depletion of CD45RO + memory T cells by staining with anti-CD45RO-PE (80 μg ml −1 ; R0843; DAKO), coated on anti-PE beads (Miltenyi). DCs were either silenced for indicated proteins or preincubated for 2 h with blocking DC-SIGN antibodies, activated for 48 h as indicated and subsequently cocultured with naive CD4 + T cells (20,000T cells/5,000 DCs) in the presence of 10 pg ml −1 Staphylococcus aureus enterotoxin B (Sigma) and after 5 days, further cultured with 10 U ml −1 IL-2 (Chiron). Resting cells were restimulated after 12–16 days with 100 ng ml −1 PMA (Sigma) and 1 μg ml −1 ionomycin (Sigma) for 6 h, the last 4 h in the presence of 10 μg ml −1 brefeldin A (Sigma) and analysed by flow cytometry for intracellular cytokine expression by staining with APC-conjugated rat anti-IL-4 (1:25; MP4-25D2; BD) and FITC-conjugated mouse anti-IFN-γ (1:5; 25723.11; BD). DCs primed with 10 ng ml −1 LPS plus 1,000 U ml −1 IFN-γ (U-CyTech) or 1 μM PGE 2 (Sigma) were used as positive controls for T H 1 and T H 2 differentiation, respectively. Statistical analysis Statistical analyses were performed on the data using the Student’s t -test for paired observations. Statistical significance was set at P <0.05. How to cite this article : Gringhuis, S. I. et al. Fucose-specific DC-SIGN signalling directs T helper cell type-2 responses via IKKε- and CYLD-dependent Bcl3 activation. Nat. Commun. 5:3898 doi: 10.1038/ncomms4898 (2014).